Dynamics of multiple phases in a colossal-magnetoresistive manganite as revealed by dielectric spectroscopy Electronic phase separation is one of the key features in correlated electron oxides. The coexistence and competition of multiple phases give rise to gigantic responses to tiny stimuli producing dramatic changes in magnetic, transport and other properties of these compounds. To probe the physical properties of each phase separately is crucial for a comprehensive understanding of phase separation phenomena and for designing their device functions. Here we unravel, using a unique p–n junction configuration, dynamic properties of multiple phases in manganite thin films. The multiple dielectric relaxations have been detected and their corresponding multiple phases have been identified, while the activation energies of dielectric responses from different phases were extracted separately. Their phase evolutions with changing both temperature and applied magnetic field have been demonstrated by dielectric response. These results provide a guideline for exploring the electronic phase separation phenomena in correlated electron oxides. The family of correlated electron oxides, such as perovskite manganites exhibiting colossal magnetoresistance, has attracted great interest in the last decades due to their exotic electronic, magnetic and structural properties [1] , [2] . One of the most interesting properties of these materials is the spontaneous phase separation between different electronic/magnetic states [1] , [3] . This sort of phase separation is a common characteristic of many correlated electron oxides, originating from the strong coupling between lattice, charge, orbital and spin degrees of freedom. The electronic phase separation has been revealed at first by magnetic and electric-transport characterization and verified consequently by a variety of structural probes, such as X-ray and neutron diffraction measurements [3] , [4] , [5] . Recently, studies using microscopies have provided us with the real space image of phase separation in correlated electron oxides [3] , [6] . Nevertheless, knowledge of dynamic transport in multiple phases is lacking up to now, although it is quite important both for understanding of underlying physics as well as promising applications [1] . It has been revealed that the microscopic phases have linear dimensions on the order of ten to several hundred nanometres and are distributed over the system almost randomly [3] , [4] , [5] . The small size and random distribution of multiple phases obstruct us to explore them separately in detail. One of the possible probes for revealing their respective dynamic transport properties is dielectric spectroscopy, as described in this paper. Recently, several works have been devoted for study of dielectric properties in correlated electron oxides and the close relation has been revealed between dielectric response and electrical transport properties [7] , [8] , [9] , [10] , [11] , [12] , [13] , [14] , [15] . Most of these dielectric measurements have been done for bulk materials. For thin films, it is more difficult to obtain the dielectric response due to the current leakage problem. Moreover, except intrinsic dielectric response of correlated electron oxides, several reports raised the concern that the dielectric behaviour includes extrinsic interface effect [14] , [15] , [16] , [17] . To avoid this contact problem, inserting an insulator layer into the measurement circuit has been adopted, but it makes the whole system more complicate [8] , [16] . In this paper, a p–n junction configuration [18] , [19] has been designed for dielectric response measurement of complex oxide thin films. With help from the depletion layer of junctions, the dynamic transport properties of multiple phases could be resolved separately. Electrical transport of manganite-based junctions As a typical phase-separated complex oxide, Pr 1− x (Ca 1− y Sr y ) x MnO 3 ( x =0.45 and y =0.25; PCSMO) was studied here in which the value of x and y were chosen so that the compound may position in the bicritical region, that is, between the ferromagnetic-metallic and the charge/orbital-ordered states, of the electronic phase diagram [20] . Near this bicritical point, the PCSMO crystal shows coexistence and competition of the two phases, which is sensitive to external stimuli [21] . In addition to this sample, the half-doped Pr 0.5 Ca 0.5 MnO 3 (PCMO) with very rigid charge-ordered (CO) state and the metallic La 0.65 Sr 0.35 MnO 3 (LSMO) have also been examined as the references [22] . With epitaxially grown manganite films (~40 nm in thickness) on n -type Nb-doped (0.01 wt%) SrTiO 3 substrates (Nb:STO), p–n junctions were built for PCMO and PCSMO samples, while a Schottky junction for metallic LSMO sample, as shown in Fig. 1a,b . The temperature dependence of in-plane dc transport properties of the three manganite films measured in selected external magnetic fields is presented in Fig. 1c . Without magnetic field, the PCMO and PCSMO films are insulating while LSMO is metallic in the whole measurement temperature range. The CO transition temperature T CO for PCMO film is above room temperature and its CO state is quite stable even at a high-magnetic field of 12 T ( Fig. 1c ). On the other hand, for PCSMO film with T CO around 205 K, the CO state collapses when the applied field exceeds 2.5 T, and a subsequent insulator–metal (I–M) transition occurs. 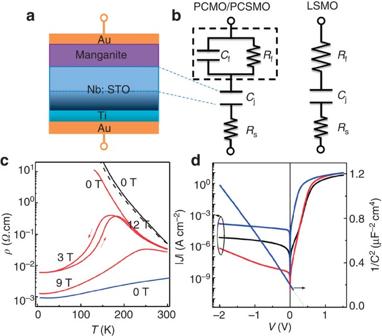Figure 1: Schematics and properties of junctions. (a) Junction configuration and (b) equivalent circuits for PCMO(PCSMO)/Nb:STO and LSMO/Nb:STO junctions. (c) Temperature dependence of in-plane resistivities for PCMO, PCSMO and LSMO films under various external magnetic fields. The arrows indicate the direction of temperature variation. The dashed line was used to present theρ–Tof PCMO film measured at 12 T field for clarity. (d) Current density–voltage (left axis) relations for three junctions and capacitance–voltage (right axis) characteristics for LSMO junction measured at 300 K. The dashed line is the extrapolation of liner fitting for1/C2−Vcurve of LSMO junction with the intercept on voltage axis ~0.38 V. In bothcandd, the black, red and blue curves present the data for PCMO, PCSMO and LSMO samples, respectively. Here PCMO, PCSMO, LSMO and Nb:STO stand for Pr0.5Ca0.5MnO3, Pr0.55(Ca0.75Sr0.25)0.45MnO3, La0.65Sr0.35MnO3and Nb-doped (0.01 wt%) SrTiO3. Figure 1: Schematics and properties of junctions. ( a ) Junction configuration and ( b ) equivalent circuits for PCMO(PCSMO)/Nb:STO and LSMO/Nb:STO junctions. ( c ) Temperature dependence of in-plane resistivities for PCMO, PCSMO and LSMO films under various external magnetic fields. The arrows indicate the direction of temperature variation. The dashed line was used to present the ρ–T of PCMO film measured at 12 T field for clarity. ( d ) Current density–voltage (left axis) relations for three junctions and capacitance–voltage (right axis) characteristics for LSMO junction measured at 300 K. The dashed line is the extrapolation of liner fitting for 1/C 2 −V curve of LSMO junction with the intercept on voltage axis ~0.38 V. In both c and d , the black, red and blue curves present the data for PCMO, PCSMO and LSMO samples, respectively. Here PCMO, PCSMO, LSMO and Nb:STO stand for Pr 0.5 Ca 0.5 MnO 3 , Pr 0.55 (Ca 0.75 Sr 0.25 ) 0.45 MnO 3 , La 0.65 Sr 0.35 MnO 3 and Nb-doped (0.01 wt%) SrTiO 3 . Full size image At the interface of the manganite/Nb:STO junctions, depletion layers are formed due to the diffusion of carries between manganites and Nb:STO [19] , [23] . The removal of free charge carriers in a depletion layer with a thickness of W d ( Fig. 1a ), leaving none to carry a current, results in an excellent insulator region working as a coupling capacitor to manganites ( Fig. 1b ). The carrier density of manganite films ( n p ~10 22 cm −3 ) are much higher than that in Nb:STO ( n n ~10 17 cm −3 ) and then ε p n p ≫ ε n n n in which ε p ( ε n ) are the static dielectric constants in p ( n )-layer. As a consequence, the depletion layers of these junctions are almost all located at the Nb:STO side according to the abrupt junction model [23] . In Fig. 1d , the current density–voltage ( J–V ) relations of junctions show good rectification, indicating the good insulator behaviour of depletion layer in Nb:STO. Following this scenario, the built-in potentials ( qV bi ) of these junctions were derived from 1/ C 2 −V curves as shown in the Fig. 1d ; 0.88, 0.83 and 0.38 eV for PCMO, PCSMO and LSMO samples, respectively. Dielectric spectroscopies of manganite-based junctions In the junction geometry, the manganite films are arranged in series with a capacitance of junction C j . As schematically shown in Fig. 1b , the metallic LSMO film has a role of a series resistor in the circuit. For PCMO and PCSMO cases, however, the manganite films can be modelled as a capacitor ( C f ) with a parallel resistor ( R f ), both connected in series to larger C j . With this configuration, the dielectric properties of manganite films can be elucidated by analysing the dielectric properties of the whole junction setup. The frequency-dependent complex capacitance C *( ω ) has been measured for three samples with a capacitive technique [7] , [16] at temperatures between 8 and 300 K. The complex dielectric spectrum is expressed as C *( ω )= C′ ( ω )− iC″ ( ω ), where C′ ( ω ) and C″ ( ω ) are the real and imaginary parts of the capacitance, respectively. Typical results for PCMO and PCSMO samples are shown in Fig. 2 . For the metallic LSMO sample, dielectric response is dominated by C j of the depletion layer in Nb:STO and has nearly no frequency dependence in a whole frequency window (10 2 ~10 6 Hz; see Supplementary Fig. S1 ). In contrast to the LSMO case, dielectric relaxation behaviours are clearly observed in both PCMO and PCSMO samples. The C″ ( ω ) has a loss peak at a specific frequency, which shifts exponentially to higher frequencies with increasing temperature; this is the characteristic of Debye-like relaxation with a thermally activated relaxation rate. The frequency of the loss peak ( f p ) is related to a relaxation time as τ p =1/2 πf p 1/ ω p . 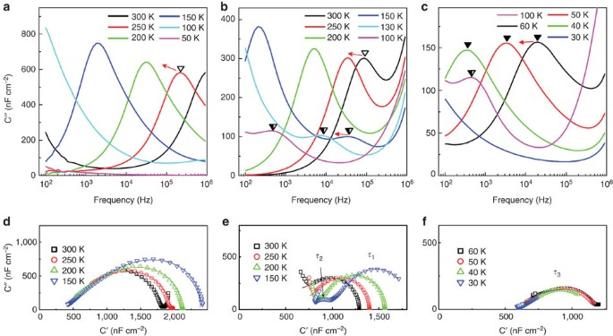Figure 2: Dielectric relaxation characteristics of junctions. (a–c) Frequency dependence of imaginary (C″) part of complex capacitances at various temperatures for manganite films; (a) PCMO, (b) and (c) PCSMO. Blank, half-filled and filled triangles indicate different loss peaks ofC″(relaxationτ1,τ2andτ3, respectively). Red arrows indicate the movement of loss peaks with decreasing temperature. (d–f) The corresponding Cole–Cole plots (C′versusC″); (d) PCMO, (e) and (f) PCSMO. The solid lines are fitting results according to the Davidson–Cole model (see text). The Davidson–Cole parameterβobtained from fitting results is ~0.5 for PCMO. For PCSMO, it is about 0.85 for relaxationτ1, about 1 for relaxationτ2and as small as 0.43 for relaxationτ3. The labelsτ1,τ2andτ3ineandfindicate the corresponding arcs in Cole–Cole plots for different relaxationτ1,τ2andτ3, respectively. Figure 2: Dielectric relaxation characteristics of junctions. ( a – c ) Frequency dependence of imaginary ( C″ ) part of complex capacitances at various temperatures for manganite films; ( a ) PCMO, ( b ) and ( c ) PCSMO. Blank, half-filled and filled triangles indicate different loss peaks of C″ (relaxation τ 1 , τ 2 and τ 3 , respectively). Red arrows indicate the movement of loss peaks with decreasing temperature. ( d – f ) The corresponding Cole–Cole plots ( C′ versus C″ ); ( d ) PCMO, ( e ) and ( f ) PCSMO. The solid lines are fitting results according to the Davidson–Cole model (see text). The Davidson–Cole parameter β obtained from fitting results is ~0.5 for PCMO. For PCSMO, it is about 0.85 for relaxation τ 1 , about 1 for relaxation τ 2 and as small as 0.43 for relaxation τ 3 . The labels τ 1 , τ 2 and τ 3 in e and f indicate the corresponding arcs in Cole–Cole plots for different relaxation τ 1 , τ 2 and τ 3 , respectively. Full size image In PCMO sample with the CO state, only one kind of loss peak can be discerned in our frequency window as marked by blank triangles in Fig. 2a . In PCSMO, however, the situation is quite different. As shown in Fig. 2b , there is discerned one loss peak (defined as τ 1 ) at high temperatures and the peak position moves to the low f region when the temperature decreases. Below 170 K, another weaker loss peak (defined as τ 2 ) emerges at higher f region as marked by half-filled triangles in Fig. 2b . With further decreasing temperature, the third relaxation τ 3 (marked by filled triangles) comes to the present measurement window as shown in Fig. 2c . Similarly to τ 1 , the peak positions of τ 2 and τ 3 shift to lower f region with decreasing temperature. It is interesting to find that the magnitude of loss peaks τ 3 is higher than that of τ 2 and smaller than that of τ 1 . The main loss peak τ 1 corresponds to the relaxation process of the main phase in PCSMO sample and its magnitude is similar to that of PCMO sample. To the contrary, the additional relaxations, τ 2 and τ 3 , originate from the phase separation of the manganite film, as will be discussed in detail later. Figure 2d–f present the corresponding Cole–Cole plots ( C′ versus C″ ) of PCMO and PCSMO samples. These experimental data provide a clear evidence that the complex capacitance spectra C *( ω ) of these two samples largely deviate from the simple Debye model (half circle). The physical processes of these deviations, manifested by broader and asymmetric shapes of the absorption term C″ of the spectra, are often described by Davidson–Cole model [24] , Here C HF ( C LF ) is the high (low) frequency limit of the capacitance, ω=2πf the angular frequency, τ the relaxation time, and β the Davidson–Cole parameter. All the C′ versus C″ curves can be well fitted with the Davidson–Cole model and the fitting results are shown by solid lines in Fig. 2 . Interestingly, we found that the parameter β for a specific relaxation process is almost constant against temperature variation, whereas its values are different for different relaxations. It is around 0.5 for PCMO at all temperatures. For PCSMO, it is about 0.85 for relaxation τ 1 , about 1 for relaxation τ 2 , and as small as 0.43 for relaxation τ 3 . The deviation of β from 1 indicates the distribution of multiple relaxation times in these strong-correlated oxides [24] . In the present junction configuration, the total capacitance C can be given approximately by 1/ C =1/ C j +1/ C f . Because of large dielectric constant in Nb:STO crystal, especially at low temperatures (~10 3 at 100 K) [25] , C j is much larger than C f , therefore the contribution from C f is dominant in the measured C -value. As shown by Cole–Cole plots in Fig. 2d–f , the variation of C HF and C LF can reflect the change of dielectric properties of samples. In PCMO sample, as shown in Fig. 2d , the C LF increases with decreasing of temperature while the C HF is almost temperature independent. We simulated C *( ω ) results by using an equivalent circuit and Barrett's law [26] for dielectric properties of Nb:STO-depletion layer C j ( Supplementary Figs S2 and –S3 ). The simulation results are consistent with this premise and the dielectric properties of manganite films could be deduced from the measured C *( ω ) spectroscopy. It was found that the static dielectric constants ε r of PCMO and PCSMO films are 39 and 22 at room temperature, respectively. The ε r of PCMO film is almost temperature independent, while the ε r of main phase in PCSMO film increases with decreasing of temperature and it reaches around 27 at T =150 K, as derived from variation of both C HF and C LF ( Fig. 2e ). In Fig. 2f , on the other hand, both C HF and C LF are temperature independent for the relaxation τ 3 . It indicates the temperature insensitivity of dielectric strength of τ 3 , which may be correlated to the ferromagnetic metal (FMM) phase involved in PCSMO film ( vide infra ). 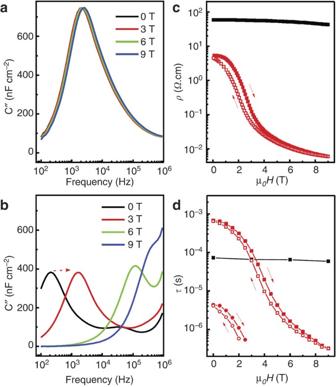Figure 3: Magnetic field dependence of dielectric relaxations. Frequency dependence ofC″under various magnetic fields for (a) PCMO and (b) PCSMO samples measured atT=150 K. Red dashed arrows inbindicate the movement of loss peaks with increasing magnetic field. (c) Magnetic field dependence of resistivity for PCMO (black) and PCSMO (red) films measured atT=150 K. (d) Magnetic field dependence of relaxation timeτfor PCMO (black) and PCSMO (red) junctions measured atT=150 K. The red curves indwith squares and circles present results for relaxationτ1andτ2of PCSMO junction, respectively. In bothcandd, the red arrows indicate the scan direction of magnetic field. Magnetic field effect on dielectric spectroscopies Figure 3a,b shows the external magnetic field effect on the dielectric responses of PCMO and PCSMO samples measured at 150 K. It is found that PCSMO shows a huge magneto-capacitive effect, while PCMO with the CO state is resistant to magnetic field. The relative magnetocapacitance C / C of PCSMO can reach 46% with a magnetic field of 3 T. Moreover, the magnetic field can shift the main loss peak of C″ ( ω ) for PCSMO film to higher frequency region, which corresponds to a tendency of a faster relaxation, for example, the peak f p ( τ p ) from 2.7×10 2 Hz (6.7×10 −4 s) to 4.8×10 5 Hz (3.3×10 −7 s) on application of 9 T field. The field sensitive/insensitive dielectric relaxations in PCSMO and PCMO are similar to the respective magnetoresistance features as shown in Fig. 3c,d . Recently, it was reported that the dc magnetoresistance with help from Maxwell–Wagner (MW) effect could contribute to the magnetocapacitance, especially in the materials with heterogeneous components [17] , [27] . In our junction configuration, the resistance of a manganite film with 40 nm (~10 −7 Ω ) is quite smaller than the value, which can be resonant with capacitance of the depletion layer ( C j ~10 −10 F) in measurement window (see Supplementary Methods ). Moreover, the asymmetric relaxation behaviour ( β <1) is not favourable for a simple MW model. Therefore, the suitable equivalent circuit for our junctions should be much more complicated if the dielectric relaxations observed here originate from the MW effect. Another possible origin for these dielectric relaxations is the contribution from small polarons in manganite films [2] , [9] , [10] . From this viewpoint, the similar temperature/magnetic field dependences for relaxation time τ and dc resistance observed here indicate the dominant role of polaronic charge carriers in both ac dielectric and dc electrical transport properties. Figure 3: Magnetic field dependence of dielectric relaxations. Frequency dependence of C″ under various magnetic fields for ( a ) PCMO and ( b ) PCSMO samples measured at T =150 K. Red dashed arrows in b indicate the movement of loss peaks with increasing magnetic field. ( c ) Magnetic field dependence of resistivity for PCMO (black) and PCSMO (red) films measured at T =150 K. ( d ) Magnetic field dependence of relaxation time τ for PCMO (black) and PCSMO (red) junctions measured at T =150 K. The red curves in d with squares and circles present results for relaxation τ 1 and τ 2 of PCSMO junction, respectively. In both c and d , the red arrows indicate the scan direction of magnetic field. 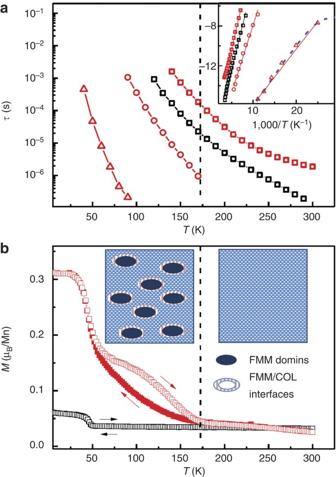Figure 4: Activation energies of dielectric relaxation processes in phase-separated manganites. (a) Temperature dependence of relaxation timeτfor PCMO (black) and PCSMO (red). The red curves with squares, circles and triangles present data forτ1,τ2andτ3of PCSMO, respectively. The inset shows Arrhenius plot of relaxation times. The solid lines in inset figure are fitting results based on Arrhenius law. The deduced activation energies for relaxationτ,τ1,τ2andτ3are 150, 160, 120 and 50 meV, respectively. The blue dotted line is fitting result forτ3based on the combined equationτ−1=τT−1+τ0−1exp(−Ea/kBT). (b) Temperature dependence of magnetization for PCMO (black) and PCSMO (red) films measured under μì0H=0.05 T. Arrows indicate the temperature scan directions. The insets schematically represent the coexistence of multiple phases in PCSMO sample. The solid ellipses and vertically patterned rings stand for ferromagnetic metal (FM) domains and interfaces between FM and charge-ordered insulator (COI) domains, respectively. Full size image Multiple phases Figure 4a presents the relaxation time τ as a function of temperature for both PCMO and PCSMO samples. Clearly, for PCSMO film three kinds of relaxations τ 1 , τ 2 and τ 3 emerge successively into the measurement window, with decreasing of temperature. In PCMO, on the other hand, only one kind of relaxation can be observed in the present measurement window. Generally, the relaxation time τ is thermally activated and its temperature dependence can be described by Arrhenius law [7] , where E a is the activation energy and k B the Boltzmann constant. The inset of Fig. 4a shows the Arrhenius plot of τ for both PCMO and PCSMO samples and the solid lines are the fitting results according to equation (2). The activation energy E a for PCMO is about 150 meV, while they are 160, 120 and 50meV for the τ 1 , τ 2 and τ 3 in PCSMO sample, respectively. To get an insight into the origin of these multiple dielectric relaxations, we refer to the temperature dependence of the dc magnetization ( M–T ) for PCMO and PCSMO samples (in a static field of 500 Oe) as shown in Fig. 4b . For PCMO with the CO state, the magnetizations in field-cooled and field-cool-field-warm (FCFW) processes are relatively small and coincident with each other. As for the phase-separated PCSMO, a kink-like feature appears at around 170 K in FCFW process. Blow this temperature ( T irr ), the FCFW and field-cooled M – T curves split. Further measurements done in higher magnetic fields show that the T irr increases with increasing field (not shown). This bifurcation behaviour indicates the formation of FMM micro-domains and the resultant coexistence of the CO-FMM phases in PCSMO below T irr [12] , [21] . On the basis of these results, we speculate the origin of the multiple dielectric relaxations in PCSMO thin film as follows. The polaronic charge carriers in major phase, that is, a paramagnetic state for T >205 K and a CO state for T <205 K, contributes to the main relaxation τ 1 with a large amplitude of loss peak and a large E a . When T < T irr , the FMM micro-domains emerge and the internal and external charger transports of those domains contribute to the relaxation τ 3 with a small E a . At the boundaries between FMM domains and CO background, build-up of charges occur (MW effect [27] ), giving rise to the relaxation τ 2 with a smallest loss peak, a middle E a and β =1. Actually, the T irr is coincident with the onset temperature of relaxation τ 2 as shown by the dashed lines in Fig. 4a,b . Figure 4: Activation energies of dielectric relaxation processes in phase-separated manganites. ( a ) Temperature dependence of relaxation time τ for PCMO (black) and PCSMO (red). The red curves with squares, circles and triangles present data for τ 1 , τ 2 and τ 3 of PCSMO, respectively. The inset shows Arrhenius plot of relaxation times. The solid lines in inset figure are fitting results based on Arrhenius law. The deduced activation energies for relaxation τ , τ 1 , τ 2 and τ 3 are 150, 160, 120 and 50 meV, respectively. The blue dotted line is fitting result for τ 3 based on the combined equation τ −1 = τ T −1 +τ 0 −1 exp(− E a / k B T ). ( b ) Temperature dependence of magnetization for PCMO (black) and PCSMO (red) films measured under μì 0 H =0.05 T. Arrows indicate the temperature scan directions. The insets schematically represent the coexistence of multiple phases in PCSMO sample. The solid ellipses and vertically patterned rings stand for ferromagnetic metal (FM) domains and interfaces between FM and charge-ordered insulator (COI) domains, respectively. Full size image We now can figure out the evolution of the phase separation under the external magnetic fields in PCSMO. As shown in Fig. 3d , the relaxation time of τ 1 is about 6.7×10 −4 s with E a ~160 meV in zero field at 150 K. With increasing magnetic field, it decreases slowly at first and then drops rapidly around 3.5 T. At 9 T, it is reduced down to 3.3×10 −7 s, which corresponds to a small activation energy of E a ~60meV if the preexponential term τ 0 remains unchanged. This energy scale is quite close to the activation energy of the relaxation τ 3 that is identified as due to the low-temperature FMM phase. This result indicates that the collapse of CO state accompanies the formation of uniform FMM state in the whole PCSMO film. Incidentally, the relaxation τ 2 shifts to the higher-frequency regime to disappear out of the present measurement window ( Fig. 3d ). Similar magnetic field effects have been observed in the whole low temperature range with T <170 K. This magneto-sensitivity observed in phase-separated manganite film may serve as a basis for their further applications, such as in magneto-capacitor and magnetic sensor. For the dielectric response of these correlated electron oxides, the ac conductivity of manganite is also important and should be taken into account [11] , [12] , [15] . We studied the dielectric contribution from ac conductivities in both PCMO and PCSMO samples (see Supplementary Fig. S4 ). On the one hand, a superlinear power law behaviour has been observed at high frequency region. This superlinear power law behaviour has also been observed in bulk Pr(Ca,Sr)MnO 3 and its origin is still an open question up to now [12] . On the other hand, as shown in the inset of Fig. 4a , there is slight deviation from pure Arrhenius law of the relaxation times, especially for τ 3 in phase-separated PCSMO. It implies that there exists other contribution to the dielectric relaxation except the purely thermally activated process. We speculate that the tunnelling effect between FMM domains in phase-separated PCSMO film is also responsible for the dielectric relaxation processes especially at low temperature region. For the tunnelling process, the time constant τ T is nearly temperature independent at low temperatures [28] . A fit to the data, combining a thermal-activated model and a tunnelling contribution by τ −1 = τ T −1 +τ 0 −1 exp(− E a / k B T ), has been added to the inset of Fig. 4a . It is found that the fitting results are much better than that with pure Arrhenius law. The time constant for tunnelling process τ T is about 9×10 −4 s and the thermal activation energy E a is ~53 meV, which is a little bit larger than that from pure Arrhenius case. These results indicate the ability of this junction configuration to reveal the transport properties in correlated electron oxides. In summary, we studied the phase separation of colossal-magnetoresistive manganite thin films using dielectric spectroscopy with a unique junction configuration. It was found that the depletion layer in Nb:STO can act as isolation layer for exploration of dielectric properties of manganite thin films. The multiple dielectric relaxations have been detected in the manganite thin film with the phase separation between the COI and FMM states. The dynamics of multiple phases and their boundaries have been deduced separately from temperature- and magnetic-field-dependent variations of the dynamic capacitance spectra. Such dielectric spectroscopy will find a broad application in the study of phase separation issues for versatile correlated-electron systems. Sample preparation The Pr 0.55 (Ca 0.75 Sr 0.25 ) 0.45 MnO 3 (PCSMO) thin films were grown on (110) surface of Nb-doped (0.01 wt%) SrTiO 3 substrates (Nb:STO). The LSMO and PCMO thin films were grown on Nb:STO (001) substrates. The LSMO (001) film with a small strain effect from the substrate shows a ferromagnetic metallic state in a whole measurement temperature range, whereas half doped PCMO (001) film is a rigid insulator with the CO state, which is stabilized by tensile strain from the substrate [22] . All these manganite films were grown by pulsed laser deposition. With epitaxial growth of the manganite films on n -type Nb:STO, junctions were built. For J–V and C–V measurements along perpendicular direction, these junctions were patterned into mesa-structure (400×600 μm 2 for PCSMO, 200×200 μm 2 for LSMO and PCMO) using a photolithographic technique. The conditions for film growth and device fabrication have been published elsewhere [18] , [19] . Electrical transport and dielectric measurements The magnetization of the sample was measured by a SQUID magnetometer (Quantum Design MPMS). The capacitances of samples were investigated at intermediate frequencies (10 2 < f <10 6 Hz) in a temperature range of 8–300 K with a precision LCR metre (Agilent, E4980A). The J–V behaviour was characterized by a precision semiconductor parameter analyzer (Agilent, 4156C). For both capacitance and J–V measurements, triaxial BNC cables were used in a cryostat equipped with a superconducting magnet. How to cite this article: Sheng, Z. et al . Dynamics of multiple phases in a colossal-magnetoresistive manganite as revealed by dielectric spectroscopy. Nat. Commun. 3:944 doi: 10.1038/ncomms1943 (2012).